Surface tension and contact with soft elastic solids The Johnson–Kendall–Roberts theory is the basis of modern contact mechanics. It describes how two deformable objects adhere together, driven by adhesion energy and opposed by elasticity. Here we characterize the indentation of glass particles into soft, silicone substrates using confocal microscopy. We show that, whereas the Johnson–Kendall–Roberts theory holds for particles larger than a critical, elastocapillary lengthscale, it fails for smaller particles. Instead, adhesion of small particles mimics the adsorption of particles at a fluid interface, with a size-independent contact angle between the undeformed surface and the particle given by a generalized version of the Young's law. A simple theory quantitatively captures this behaviour and explains how solid surface tension dominates elasticity for small-scale indentation of soft materials. Contacts between solid surfaces are found throughout nature and have important roles in almost every scientific field from physics [1] , [2] , [3] and biology [4] , [5] to astrophysics [6] , [7] and meteorology [8] , [9] . From an engineering perspective, an understanding of contacts is essential to control friction and adhesion [10] , [11] , [12] , [13] , [14] , [15] . The Johnson–Kendall–Roberts (JKR) theory is the basis of modern contact mechanics [13] . It predicts the form of contacts between soft, adhesive surfaces by balancing adhesion energy, which favours contact, against elastic energy, which opposes deformation. Whereas the JKR theory was originally developed to describe macroscopic contacts, it has been widely applied to microscopic systems [2] , [16] , [17] , [18] and to rough surfaces where contact is dominated by microscopic asperities [10] , [19] , [20] . Here we show that the JKR theory can break down at these microscopic lengthscales because of the effects of solid surface tension. Recent experiments have illustrated that solid surface tension, Υ sv , can have a dominant role in the behaviour of soft materials [21] , [22] , [23] , [24] , [25] , [26] , [27] . Solid surface tension drives a rippling instability in soft, elongated structures [28] . It smooths out sharp features, limiting the resolution of lithography in gels and elastomers [29] , [30] , [31] . It also determines the wavelength of surface creases and ripples in a compressed gel [32] , [33] . These solid capillary effects become significant below a critical elastocapillary lengthscale, L [28] , [31] . The basic physics is highlighted by the following argument: consider a surface with a sinusoidal corrugation of wavelength λ . Surface tension acts to flatten the surface, with a stress that scales like Υ sv / λ 2 . On the other hand, elastic forces will resist this deformation with a restoring stress that scales like E / λ , where E is Young's modulus. When , solid surface tension overpowers elastic restoring forces and flattens the surface. Solid capillarity can be seen at the micron-scale for gels, at the nanometre-scale for elastomers and is unimportant for harder materials such as glass [23] , [24] , [34] , [35] . This scaling suggests that solid surface tension, ignored by JKR, may dominate small contacts with soft solids. Here we show that the JKR theory fails for small contacts on soft materials because it ignores solid surface tension. Instead, small contacts are described by a generalization of Young's law for liquid wetting on stiff solids [36] . Our results have important implications for any processes involving small contacts on soft materials including elastomers, gels, tissues and cells. For example, JKR may not be appropriate for interpreting nanoindentation or atomic force microscopy (AFM) data for soft materials. Furthermore, solid surface tension can have an impact on adhesion and friction of rough and hierarchical surfaces. Measuring indentation We tested the validity of the JKR theory by using confocal microscopy to measure the spontaneous indentation of hard, silica microspheres into soft, sticky, flat, silicone substrates. We varied the particle size (3–30 μm radii) and substrate stiffnesses ( E =3, 85, 150 and 500 kPa) and compared the resulting indentation profiles with theoretical predictions. Example of surface profiles under 15 μm spherical particles for three different stiffnesses are shown in Fig. 1 . In each profile, the particle indents the substrate, with the indentation depth decreasing with substrate stiffness. The measured indentation is entirely because of substrate–particle adhesion—Hertz theory predicts that the weight of the particles causes sub-nanometre indentations [37] . The substrate surface is also pulled up, adhering to the particle sides and creating a ridge at the contact line. The clearest ridge appears on the intermediate 85 kPa surface. For the 3 kPa substrate, the surface outside the particle is surprisingly flat, despite very large deformations under the bead—reminiscent of a particle adsorbed at a liquid surface [36] . Despite this ‘liquid-like' behaviour of the gel, it exhibits no plastic deformation at these strains [38] , [39] , [40] , as shown by rheology in Supplementary Fig. S6 . Note that for the softest substrates, we could not image the contact line completely, as the contact line is on the top half of the bead and the objective is below the substrate. Qualitatively, similar profiles are seen for all 110 particles examined—each shown in Supplementary Figs S1–S4 . 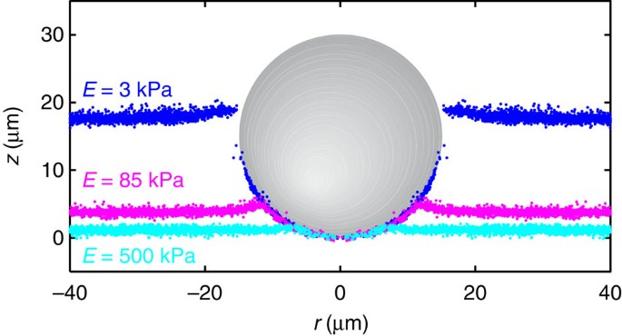Figure 1: Surface indentation profiles upon adhesion. Coloured data show surface profiles of silicone substrates upon adhesion to spherical silica particles of radii 15 μm. No external forces are applied to the particles except for their weight, which causes negligible indentation. Substrate stiffnesses are 3 kPa (blue), 85 kPa (magenta) and 500 kPa (cyan). Figure 1: Surface indentation profiles upon adhesion. Coloured data show surface profiles of silicone substrates upon adhesion to spherical silica particles of radii 15 μm. No external forces are applied to the particles except for their weight, which causes negligible indentation. Substrate stiffnesses are 3 kPa (blue), 85 kPa (magenta) and 500 kPa (cyan). Full size image We extracted the indentation d and contact radii a of the particles from the surface profiles. As shown in Fig. 2 , d is the depth of the bottom of the particle relative to the undeformed substrate surface, and a is the radius of the circular contact line. 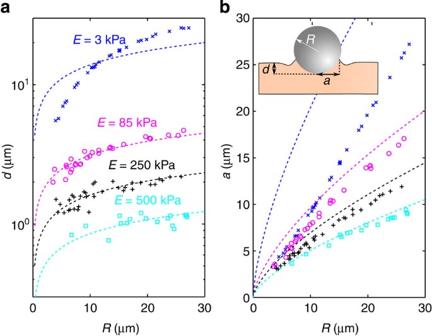Figure 2: Effects of stiffness and size. (a) Indentation depth versus particle radius and (b) contact radius versus particle radius for silica microspheres on silicone substrates of differing stiffnesses. Points show measured data for substrates with stiffness 3 kPa (blue), 85 kPa (magenta), 250 kPa (black) and 500 kPa (cyan). Dashed curves are the best-fit predictions from the JKR theory. Inset: schematic showing the definitions of indentation,d, contact radius,a, and particle radiusR. Figure 2a shows d versus particle radius, R , for different substrate stiffnesses. Indentation increases with particle size and decreases with substrate stiffness. Figure 2b shows the contact radii for the same experiments. Contact radii similarly increase with particle size and decrease with substrate stiffness. Figure 2: Effects of stiffness and size. ( a ) Indentation depth versus particle radius and ( b ) contact radius versus particle radius for silica microspheres on silicone substrates of differing stiffnesses. Points show measured data for substrates with stiffness 3 kPa (blue), 85 kPa (magenta), 250 kPa (black) and 500 kPa (cyan). Dashed curves are the best-fit predictions from the JKR theory. Inset: schematic showing the definitions of indentation, d , contact radius, a , and particle radius R . Full size image Comparison with the JKR theory These results reveal significant limitations of the JKR theory. The JKR theory applies for particles on elastic substrates when d is much bigger than intermolecular distances [41] , [42] and clearly should be applicable to our data. In the absence of an external load, it predicts an indentation , and contact radius a =[9π W (1– ν 2 )/2 E ] 1/3 R 2/3 . Here ν is the substrate's Poisson ratio and the adhesion energy is defined as W = γ sv + γ pv − γ sp , the change in interfacial energy on particle adhesion, per unit area. Subscripts s, p and v indicate the soft substrate, hard particle and vapour, respectively. Silicone is nearly incompressible; therefore, ν=1/2 and the only unknown is the adhesion energy W —expected to be nearly the same for all the substrates. We fit the indentation to the JKR prediction for each of the substrates, as shown in Fig. 2a . For the three stiffer substrates, the JKR theory agrees well with the indentation data, giving similar values of the adhesion energy: W =72, 80 and 61 mN m −1 for the 85, 250 and 500 kPa substrates, respectively. For the 3 kPa substrates, even the best-fit value of W =24 mN m −1 shows strong systematic deviation of the data from the JKR theory. Measured contact radii are compared with the JKR theory with the same values of W in Fig. 2b . Moreover, JKR agrees reasonably well with the contact radii for the three stiffest substrates, despite a small systematic overestimate of the contact radius. However, the JKR theory works for neither indentation nor contact radius when E =3 kPa. The precise conditions where the JKR theory starts to breakdown can be found by collapsing the indentation and contact radius data on a single curve. In contact mechanics theory, a and d can only depend on E and R and the interfacial tensions/energies. We expect these interfacial quantities—such as W and Υ sv —to be nearly identical for all of our silicone substrates. Then, dimensional analysis shows that Ed / W and Ea / W can only vary with ER / W , or alternatively Ea and Ed can only depend on ER . 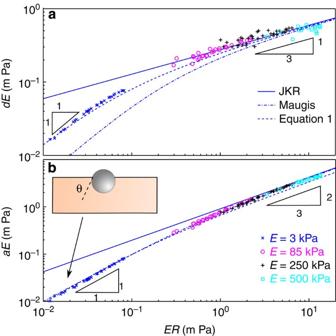Figure 3: Collapse of indentation data. (a) Indentation × Young’s modulus versus bead radius × Young’s modulus. (b) Contact radius × Young’s modulus versus bead radius × Young’s modulus. Inset: schematic of particle behaviour for. For both quantities, the data collapses on a smooth curve. The dotted line shows the best-fit JKR theory13. The dash-dotted curve shows Maugis’s extended JKR predictions43. The dashed curve is derived from equation 2. Points show measured data for substrates with stiffness 3 kPa (blue), 85 kPa (magenta), 250 kPa (black) and 500 kPa (cyan). Figure 3a,b shows the smooth collapse of the data when scaled by E . The collapsed curves show that for large beads on stiffer substrates ( m Pa), the data matches with the JKR theory with W =71 mN m −1 , the average of the adhesion energies determined earlier for the three stiffer substrates. For m Pa, there is a smooth deviation from the JKR predictions to a regime where d and a appear proportional to the particle radius. Figure 3: Collapse of indentation data. ( a ) Indentation × Young’s modulus versus bead radius × Young’s modulus. ( b ) Contact radius × Young’s modulus versus bead radius × Young’s modulus. Inset: schematic of particle behaviour for . For both quantities, the data collapses on a smooth curve. The dotted line shows the best-fit JKR theory [13] . The dash-dotted curve shows Maugis’s extended JKR predictions [43] . The dashed curve is derived from equation 2. Points show measured data for substrates with stiffness 3 kPa (blue), 85 kPa (magenta), 250 kPa (black) and 500 kPa (cyan). Full size image If JKR fails at small ER , what is the governing physics at this scale? The indentation profiles and scaling offer two important clues. First, in the small ER regime, the indentation and contact radius scale with the particle radius: . This suggests that the undeformed surface of the substrate intersects the indenting sphere at a size-independent contact angle, θ , as shown in the inset of Fig. 3b . Second, despite very large indentations, the substrates show nearly flat surfaces, as seen in Fig. 1 and Supplementary Fig. S1 . These two features, which directly contradict the predictions of JKR, are instead identical to the surface-tension-dominated behaviour of stiff particles adsorbed at a liquid surface [36] . Thus, our results suggest a crossover from elastic to capillary contacts as ER becomes smaller. We need to rule out two other causes to confirm that the small ER behaviour is because of solid surface tension. First, the JKR theory assumes a parabolic, rather than spherical, particle shape. We considered Maugis's extension of the JKR theory for large deformations [43] . Maugis's predictions are shown as dash-dotted curves in Fig. 3a,b , with W =71 mN m −1 . Even though this extension of JKR gives good agreement with the contact radii, there is a large deviation from the indentation data for small ER . Maugis’s theory also predicts qualitatively different profiles to those measured in the experiments. 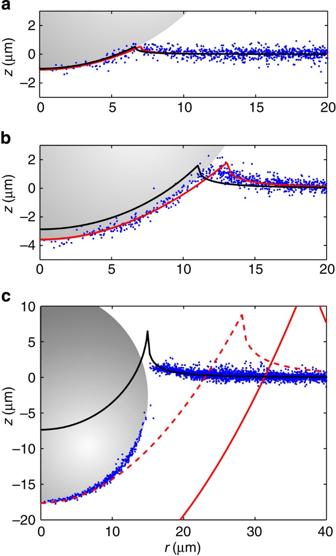Figure 4: Surface profiles compared with theory. Beads are 15 μm in radius. (a)E=500 kPa, (b)E=85 kPa, (c)E=3 kPa. The JKR theory (red curves)13and extended JKR theory (black curves)43are shown forW=71 mN m−1. Note the change in horizontal scale inc. For theE=3 kPa substrate in the JKR theory is shown withW=81 mN m−1chosen to match the particle indentation (red-dashed). Figure 4 shows the substrate profiles from Fig. 1 along with JKR and Maugis predictions with W =71 mN m −1 . For the stiffer substrates, both theories work well. However, for the soft substrate, the measured profiles differ substantially from the theoretical ones. Most obviously, Maugis’ theory predicts a sharp ridge at the contact line, which is missing in the data. The second possible reason for failure of the JKR/Maugis theory is that they only apply for linear-elastic response of the substrate. For the soft, gel substrate, deformations are clearly not small. However, we found that the gel shows a linear stress–strain relationship until over 100% shear strain (see Supplementary Fig. S6 ); therefore, Maugis’ large-deformation linear-elastic theory should give a reasonable approximation of the substrate surface profile. The large qualitative differences between experiments and theory ( Fig. 4 ) indicate that, despite possible nonlinear effects, solid surface tension is a dominant effect in flattening the surface and controlling the particle indention in the small ER regime. Figure 4: Surface profiles compared with theory. Beads are 15 μm in radius. ( a ) E =500 kPa, ( b ) E =85 kPa, ( c ) E =3 kPa. The JKR theory (red curves) [13] and extended JKR theory (black curves) [43] are shown for W =71 mN m −1 . Note the change in horizontal scale in c . For the E =3 kPa substrate in the JKR theory is shown with W =81 mN m −1 chosen to match the particle indentation (red-dashed). Full size image The particle sizes and substrate stiffnesses in which solid capillary effects arise can be calculated from a simple scaling argument. The characteristic horizontal lengthscale in the system is min min(( WR 2 / E ) 1/3 , R ), where the scaling for a comes from the JKR theory. Solid surface tension becomes important whenever this is smaller than Υ sv / E . Thus, we expect a capillary regime for . This is similar to the scaling found for theoretical predictions of nanoparticle adhesion on hard surfaces [44] . For Υ sv =30 mN m −1 (ref. 24 ) and W =71 mN m −1 , the crossover will occur when mN m −1 , consistent with the transition behaviour seen in Fig. 3 . A simple energy argument, modified from Carrillo et al. [44] explains the transition from capillary to elastic regimes. Breaking the particle adhesion process down into two stages, we first create a spherical indentation in the substrate, then we adhere the particle on the indented area. According to Hertz theory [37] , the elastic energy required to make a spherical indentation of depth d and radius of curvature R is . Indenting the substrate also stretches the surface, creating new surface area. This introduces another energy penalty, ignored by JKR, equal to the surface tension times the additional surface area. Approximating the indentation as a spherical cap in a flat plane gives U Υ = π Υ sv d 2 (see the Supplementary Discussion and Supplementary Fig. S5 for further details). Note that the surface tension (also known as surface stress), Υ sv , is not always equivalent to the interfacial energy γ sv [45] , [46] . For solids, γ sv gives the work needed to create additional surface area by cleaving, whereas Υ sv gives the work needed to create additional surface area by stretching. For fluids, γ sv =Υ sv . The final contribution to the total energy comes from adhesion of the particle to the stretched substrate. This is the term that drives indentation and is equal to W times the adhered area, U ad =−2π WRd (again, we approximate the indentation as a spherical cap in a flat plane). Thus, the total energy change upon indentation is where c is a constant to be determined. Minimizing U with respect to d , we obtain for large R , adhesion is balanced by elasticity, and we recover JKR theory with . This is shown schematically in Fig. 5a . For small R , the elastic response of the substrate falls out and adhesion is balanced by substrate surface tension, with equation 2 reducing to d = WR /Υ sv . 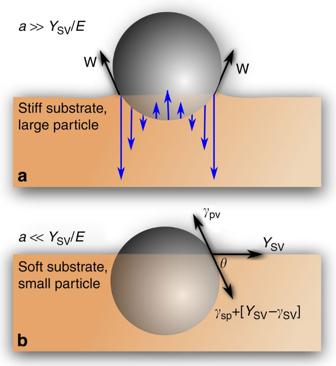Figure 5: Hard and soft contacts. (a) When the contact radius is much larger than Υsv/E, the contact is described by the JKR theory, which balances adhesion and elastic stresses (blue arrows). The surface tension contribution is negligible. (b) When the contact radius is much smaller than Υsv/E, surface tension governs contact mechanics and adhesion mimics adsorption on a fluid interface. The undeformed solid surface hits the particle at a fixed contact angle given by the generalized Young’s law in equation 3. Elastic forces are negligible. Equivalently, Figure 5: Hard and soft contacts. ( a ) When the contact radius is much larger than Υ sv / E , the contact is described by the JKR theory, which balances adhesion and elastic stresses (blue arrows). The surface tension contribution is negligible. ( b ) When the contact radius is much smaller than Υ sv / E , surface tension governs contact mechanics and adhesion mimics adsorption on a fluid interface. The undeformed solid surface hits the particle at a fixed contact angle given by the generalized Young’s law in equation 3. Elastic forces are negligible. Full size image where θ is the angle of the sphere’s surface relative to the undeformed substrate at the contact line, analogous to the contact angle in wetting. This result reduces to Young's law when the substrate has a fluid-like surface tension Υ sv = γ sv . More generally, we find that the adhesion of small spheres to soft surfaces is formally identical to the adsorption of hard particles to a fluid interface ( Fig. 5 ). Our indentation data are well described by the simple energy scaling embodied in equation 2. We use the measured value of W =71 mN m −1 and fit Υ sv =45 mN m −1 . The results are in excellent agreement with the data in Fig. 3a . The contact radius is estimated from the spherical-cap relationship . This systematically underestimates the contact radius in the elastic regime, as we ignore the adhesive ridge. Despite this, it nicely captures the transition from capillary to elastic regimes in Fig. 3b . The extracted value of Υ sv is a similar magnitude to previously measured values of Υ sv =31±5 mN m −1 (ref. 24 ). A caveat is that our scaling uses a linear-elastic approximation for the elastic energy. This does not affect the accuracy of theoretical predictions in the JKR or capillary-dominated limits. However, it may lead to inaccuracies in predictions of indentations and contact radii in the transition region, where strains are large and elastic energy is important. These results demonstrate a new technique for measuring surface stresses in soft solids by measuring particle indentations. Indentation with a large particle in the JKR regime gives the adhesion energy, W . Indentation with a small particle in the capillary regime gives the surface tension Υ sv from the relationship Υ sv = WR / d . There are currently only a few, recently developed techniques for measurement of solid surface tensions in soft surfaces. These either require imaging of surface profiles close to a droplet contact line [24] , detailed elastic models [31] or bending of elastic membranes on wetting [47] . This indentation offers a new, simpler method for dry measurement of surface tensions. The mechanical characterization of soft substrates by nanoindentation and AFM is likely very sensitive to surface tension. The curvature of an AFM tip can be just a few nanometres. There, solid surface tension will certainly affect indentations of gels and elastomers, in which the elastocapillary lengths are on the scale of tens of microns or tens of nanometres, respectively. On the other hand, the effect of solid surface tension can be reduced by submerging the substrate in a fluid that lowers its surface tension, reducing the critical lengthscale L . Note also that in the limit of very small indenters, effects such as line tension or the breakdown of continuum theory may also become important [48] . In conclusion, the JKR contact theory breaks down when contact radii are smaller than a critical elastocapillary length. In this regime, the adhesion of stiff particles to soft solids mimics the adsorption of particles at a fluid interface. Consequently, solid surface tension must be accounted for in the interpretation of AFM and nanoindentation data on a variety of soft surfaces. Our theoretical predictions match well with measured indentation depths for force-free indenters and suggest a new, straightforward method of measuring solid surface tensions via indentation. Our results should be extended to externally forced particles; whenever min , JKR or Hertz theories will not hold because of significant solid surface tension effects. Future work should consider contact between two soft solids. In that case, for small particle contacts, we anticipate similar behaviour to the wetting of a liquid droplet on an immiscible fluid substrate. Our results elucidate a fundamental difference in the contact mechanics of soft and hard materials, summarized in Fig. 5 , and may lead to novel approaches to engineering adhesion and friction. Substrate fabrication Soft adhesive substrates were created by spin-coating silicone gel and elastomer on glass slides. We prepared very soft substrates with thickness h =150 μm from a silicone gel (CY 52-276 A/B, Dow Corning). Through a combination of shear rheometry and tensile testing on an ARES-LS1 rheometer, we determined that the gel has Young's modulus E =3 kPa and Poisson’s ratio ν =0.495. The rheometry also shows a linear-elastic response to over 100% shear strain (see Supplementary Fig. S6 ). We made stiffer substrates with h =70–72 μm and with E =85, 250 and 500 kPa from a silicone elastomer (Sylgard 184, Dow Corning). The elastomer highly elastic, with rheology documented in the literature (for example, Chen et al. [49] ). Young’s moduli for the elastomer substrates were interpolated from previously reported data [50] , [51] , [52] . To image substrate topography, we covalently attached fluorescent nanobeads (40 nm carboxylated Yellow-Green Fluospheres, Invitrogen) to the substrates [53] . These covered a total area fraction of <10 −3 . To facilitate nanobead attachment, the substrates were exposed to (3-Aminopropyl)triethoxysilane vapour for 2 min. Measuring indentation profiles We quantified the deformation of substrates after adhesion to microscopic glass spheres. We distributed 3 to 30 μm radii glass spheres (Polysciences) well-apart on the substrate and recorded the positions of the underlying fluorescent nanobeads using confocal microscopy with a 60 × , NA 1.2 objective [22] , [24] . Nanobead positions were then extracted by image analysis and azimuthally collapsed to give radial surface profiles under each silica particle [24] . An example is shown in Supplementary Figs S7, S8 . From the radial profiles, we determined silica particle radii by fitting a circle through the adhered section of the substrate surface. These values agreed with particle radii measured using brightfield imaging. In total, we measured 110 particles on the four different substrate stiffnesses and ensured that substrates were much thicker than the contact radii between the particles and the substrate. How to cite this article: Style, R. W. et al. Surface tension and contact with soft elastic solids. Nat. Commun. 4:2728 doi: 10.1038/ncomms3728 (2013).